Superconductivity at the border of electron localization and itinerancy The superconducting state of iron pnictides and chalcogenides exists at the border of anti-ferromagnetic order. Consequently, these materials could provide clues about the relationship between magnetism and unconventional superconductivity. One explanation, motivated by the so-called bad metal behaviour of these materials proposes that magnetism and superconductivity develop out of quasi-localized magnetic moments that are generated by strong electron–electron correlations. Another suggests that these phenomena are the result of weakly interacting electron states that lie on nested Fermi surfaces. Here we address the issue by comparing the newly discovered alkaline iron selenide superconductors, which exhibit no Fermi-surface nesting, to their iron pnictide counterparts. We show that the strong-coupling approach leads to similar pairing amplitudes in these materials, despite their different Fermi surfaces. We also find that the pairing amplitudes are largest at the boundary between electronic localization and itinerancy, suggesting that new superconductors might be found in materials with similar characteristics. Superconductivity often occurs near a magnetic order. This is the case not only in the iron-based compounds [1] , [2] , [3] but also in heavy fermion intermetallics, organic charge-transfer salts and copper oxides. An important question that is central to these diverse classes of unconventional superconductors is whether the mechanism of their superconductivity is in a way analogous to that of conventional superconductors, with spin fluctuations replacing phonons as the glue for electron pairing, or it instead involves novel electronic states that are generated by strong electron correlations [4] . Iron-based superconductors represent a unique setting to elucidate this basic issue: their large materials parameter space provides the opportunity to understand the microscopic physics by comparing the properties across their material families. A major recent development suitable for this important characteristics is the discovery of high-temperature superconductivity in a new family of iron chalcogenides, the alkaline iron selenides K 1− x Fe 2− y Se 2 (ref. 5 ). Other related iron selenides, with K replaced in part or in entirety by Rb, Cs or Tl behave similarly [6] , [7] . The key property is that the maximum of the superconducting transition temperature ( T c ) observed in the alkaline iron selenides, above 30 K, is similar to that of their 122 iron pnictides counterpart, suggesting a commonality in the underlying mechanism for superconductivity across these systems. Compared with those of the iron pnictides, the Fermi surfaces in the alkaline iron selenides are very different. Although the former contain both electron and hole pockets, respectively, at the boundary (M) and centre (Γ) of the one-Fe Brillouin zone, only electron pockets are present in the alkaline iron selenides [8] , [9] , [10] . The weak-coupling Fermi-surface-based mechanism will operate very differently in the alkaline iron selenides compared with the iron pnictides [11] , [12] , [13] . Here we demonstrate that, by incorporating the bad metal nature of the normal state, the strong-coupling approach provides the understanding for the comparable pairing strength in the alkaline iron selenides and iron pnictides. Proximity to Mott transition We seek for the commonality between the iron chalcogenides and pnictides based on the observation that the parent compound of the alkaline iron selenides are anti-ferromagnetic insulators [6] , [14] . These insulating selenides contain Fe vacancies that are ordered in the Fe-square lattice, so that the Fe valence is kept at +2. Because of their very large ordered moment of about 3.3 μ B /Fe (refs 15 , 16 ), they are naturally considered as Mott insulators, arising through a kinetic energy reduction induced by the ordered vacancies [17] , [18] . An important question is how U / W , the ratio of a combined onsite Coulomb and Hund’s interaction to the electron bandwidth, compares with the Mott-transition threshold, U c / W . Given that a modest reduction of the kinetic energy from the parent iron pnictides to the parent alkaline iron selenides turns the system from metallic to insulating, we can infer that U / W is larger than but close to U c / W in the alkaline iron selenides, whereas smaller than but also close to U c / W in the iron pnictides. Hence, both superconductors arise out of bad metals on the verge of a Mott localization. This is illustrated in Fig. 1 showing the parent compounds of the alkaline iron selenides and iron pnictides in the vicinity of, albeit on the two sides of, the Mott transition point. Consequently, we use the Mott transition point as anchoring the regime of the phase diagram that has strong anti-ferromagnetic correlations, illustrated by the purple shading in Fig. 1 . At the Mott transition point, all the electronic excitations are incoherent. Integrating out the gapped electronic excitations gives rise to a model of localized spins with nearest-neighbour (n.n.) ( J 1 ) and next-nearest-neighbour (n.n.n.) ( J 2 ) interactions on the Fe-square lattice. In the carrier doped regime, a five-band t – J 1 – J 2 model ensues [19] , [20] , [21] . More generally, for the iron pnictides, the proximity to the Mott transition has also been supported by the bad metal behaviour of the normal state, as determined by the optical conductivity [3] and other measurements, providing the basis for strong-coupling approaches to superconductivity [19] , [20] , [21] , [22] , [23] , [24] , [25] , [26] . 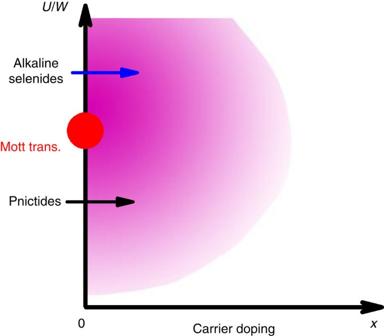Figure 1: Schematic phase diagram near a Mott transition. In this zero-temperature phase diagram, the red point located on theU/Waxis refers to the point of the Mott transition, whereas the purple shading illustrates the regime that has strong anti-ferromagnetic correlations. The parent compounds of alkaline iron selenides and iron pnictides are located in the vicinity of, albeit on the two sides of, the Mott transition. Superconductivity occurs at non-zero carrier doping, with the optimal doping located in the region indicated by the arrows. Figure 1: Schematic phase diagram near a Mott transition. In this zero-temperature phase diagram, the red point located on the U / W axis refers to the point of the Mott transition, whereas the purple shading illustrates the regime that has strong anti-ferromagnetic correlations. The parent compounds of alkaline iron selenides and iron pnictides are located in the vicinity of, albeit on the two sides of, the Mott transition. Superconductivity occurs at non-zero carrier doping, with the optimal doping located in the region indicated by the arrows. Full size image Multiorbital t – J 1 – J 2 approach We study spin singlet pairings in two such five-band t – J 1 – J 2 models, respectively, for the alkaline iron selenides and iron pnictides. The different Fermi surfaces arise from different choices of the tight-binding parameters, which are specified by the kinetic energy part of the model. The five 3 d orbitals of iron are used to correctly describe the Fermi surfaces; they are denoted by α =1,...,5, which correspond to 3 d xz , 3 d yz , , 3 d xy and (see Methods). The Fermi surface of K 1− x Fe 2− y Se 2 is shown in Fig. 2a . It comprises electron pockets only, and corresponds to an electron doping of about 15% per Fe; both have been specified in accordance with the angle-resolved photoemission spectroscopy (ARPES) measurements [8] , [9] , [10] . The electron- and hole-like Fermi pockets for the iron pnictides [27] , also with δ =15% electron doping, are displayed in Fig. 2b . The xz / yz and xy 3 d orbitals dominate the electronic states near the Fermi surfaces, as illustrated in Fig. 2c,d . We observe that, at and near zero doping ( δ =0), the ground state will be anti-ferromagnetically ordered (see below). We also note that our study focuses on the couplings in the spin sector as driving the superconductivity, although our general analysis may also have implications for the considerations in the orbital sector [26] . 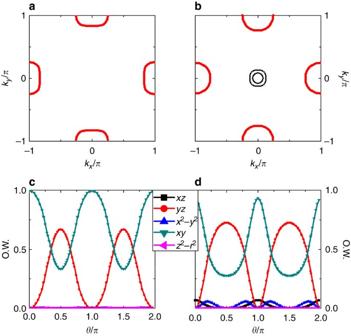Figure 2: The contrasting Fermi surfaces of K1−xFe2−ySe2and iron pnictides. aandb, respectively, show the Fermi surfaces of K1−xFe2−ySe2and iron pnictides in the extended Brillouin zone corresponding to one iron per unit cell, as obtained by using a five-orbital tight-binding model described in the Methods section, for electron dopingδ=0.15. There are only electron pockets at the M points (±π,0) and (0,±π) for K1−xFe2−ySe2. For iron pnictides, there are in addition two hole pockets near the Γ point (0,0). (c,d) The corresponding orbital weights (O.W.) on the electron pockets centred at (π,0) inaandb.θis the winding angle of the pocket with respect to its centre. The weights on the electron pocket centred at (0,π) can be obtained by interchanging thexzandyzcomponents and shiftingθbyπ/2. Figure 2: The contrasting Fermi surfaces of K 1− x Fe 2− y Se 2 and iron pnictides. a and b , respectively, show the Fermi surfaces of K 1− x Fe 2− y Se 2 and iron pnictides in the extended Brillouin zone corresponding to one iron per unit cell, as obtained by using a five-orbital tight-binding model described in the Methods section, for electron doping δ =0.15. There are only electron pockets at the M points (± π ,0) and (0,± π ) for K 1− x Fe 2− y Se 2 . For iron pnictides, there are in addition two hole pockets near the Γ point (0,0). ( c,d ) The corresponding orbital weights (O.W.) on the electron pockets centred at ( π ,0) in a and b . θ is the winding angle of the pocket with respect to its centre. The weights on the electron pocket centred at (0, π ) can be obtained by interchanging the xz and yz components and shifting θ by π /2. 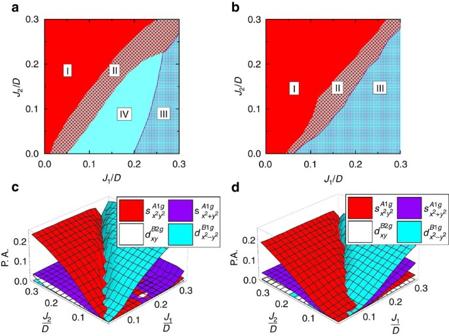Figure 3: Phase diagram and pairing amplitudes of K1−xFe2−ySe2and iron pnictides. The results presented here are for electron dopingδ=0.15.aandb, respectively, show the zero-temperature phase diagrams of K1−xFe2−ySe2and iron pnictides. Region I corresponds to an A1gstate with dominantchannel. Regions II and III mark an A1g+iB1gstate with dominantandchannels (II), and dominantandchannels (III); the phase locking occurs only at low temperatures. Region IV for K1−xFe2−ySe2is a pure B1gstate with dominantchannel. (c,d)The corresponding pairing amplitudes for thexy3d orbital of K1−xFe2−ySe2and iron pnictides. Full size image Figure 3a,b demonstrates how superconductivity in the five-band t – J 1 – J 2 is magnetically driven by the short-range J 1 – J 2 exchange interactions. Shown here, respectively, for K 1− x Fe 2− y Se 2 and iron pnictides, are the zero-temperature phase diagrams in the J 1 – J 2 plane, for 0≤ J 1 and J 2 ≤0.3 D , where D is the renormalized bandwidth. For K 1− x Fe 2− y Se 2 , the J 2 -dominated region I has A 1 g symmetry, with (cos k x cos k y ) wave being the dominant pairing component. Regions II, III and IV are primarily of the B 1 g (cos k x −cos k y ) wave character. The distinction among the three regions reflects the difference in the admixture of a small A 1 g component at zero (and low) temperatures (see Methods). This is similar to the phase diagram of the pnictides case, where the J 2 -dominated region I also is primarily A 1 g wave, and regions II and III are primarily B 1 g wave. Figure 3: Phase diagram and pairing amplitudes of K 1− x Fe 2− y Se 2 and iron pnictides. The results presented here are for electron doping δ =0.15. a and b , respectively, show the zero-temperature phase diagrams of K 1− x Fe 2− y Se 2 and iron pnictides. Region I corresponds to an A 1 g state with dominant channel. Regions II and III mark an A 1 g + i B 1 g state with dominant and channels (II), and dominant and channels (III); the phase locking occurs only at low temperatures. Region IV for K 1− x Fe 2− y Se 2 is a pure B 1 g state with dominant channel. ( c , d )The corresponding pairing amplitudes for the xy 3d orbital of K 1− x Fe 2− y Se 2 and iron pnictides. Full size image To clarify the admixture of the different pairing components, we show the evolution of the amplitudes of these components, projected onto the 3 d xy orbital, in Fig. 3c,d . Comparing the two figures clearly shows that, for the alkaline iron selenides, the dominant pairing amplitudes in the and channels are comparable to their counterparts in the iron pnictides. This is further illustrated in Fig. 4a,b , which shows the pairing amplitudes, also projected to the 3 d xy orbital, versus J 1 / D for a fixed J 2 / D =0.1. The same conclusion applies to the pairing amplitudes projected to the other 3 d orbitals, as shown in Fig. 4c,d for the case of 3 d xz /3 d yz orbitals. 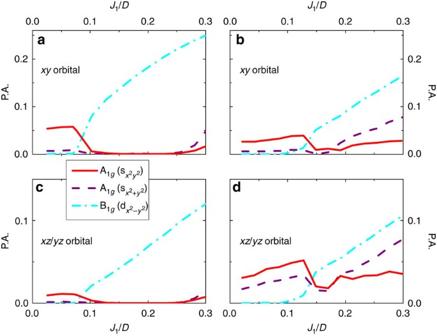Figure 4: Pairing amplitudes of K1−xFe2−ySe2and iron pnictides forxyandxz/yzorbitals. (a,b) Comparison of the competing dominant pairing amplitudes A1g, A1gand B1gfor thexy3d orbital of K1−xFe2−ySe2and iron pnictides, both for electron dopingδ=0.15 andJ2/D=0.1. (c,d) The same asaandbbut for thexz/yz3d orbitals. For K1−xFe2−ySe2the amplitude for the A1gchannel is strongly suppressed compared with the pnictides case. Correspondingly, a pure B1gstate is observed for K1−xFe2−ySe2but is absent in iron pnictides. Figure 4: Pairing amplitudes of K 1− x Fe 2− y Se 2 and iron pnictides for xy and xz / yz orbitals. ( a,b ) Comparison of the competing dominant pairing amplitudes A 1 g , A 1 g and B 1 g for the xy 3d orbital of K 1− x Fe 2− y Se 2 and iron pnictides, both for electron doping δ =0.15 and J 2 / D =0.1. ( c,d ) The same as a and b but for the xz / yz 3d orbitals. For K 1− x Fe 2− y Se 2 the amplitude for the A 1 g channel is strongly suppressed compared with the pnictides case. Correspondingly, a pure B 1 g state is observed for K 1− x Fe 2− y Se 2 but is absent in iron pnictides. Full size image Pairing amplitudes in alkaline iron selenides We therefore reach the conclusion that the pairing amplitudes in models, respectively, for the alkaline iron selenides and iron pnictides are similar for given dimensionless exchange interactions, J 1 / D and J 2 / D . This is surprising because the alkaline iron selenides lack any hole Fermi pocket and, therefore, do not possess any Fermi-surface nesting. Our result is inherent to the strong-coupling approach; here, although the details of the Fermi surfaces are important, the superconducting pairing does not require coupling between hole and electron Fermi pockets. Instead, the driving force for the pairing lies in the close-neighbour exchange interactions, J 1 and J 2 . The presence of electron pockets near the M points of the Brillouin zone is adequate to promote the cos k x cos k y A 1 g wave pairing, as well as the cos k x −cos k y B 1 g wave pairing. For similar ratios of J 1 / D and J 2 / D , the corresponding pairing amplitude is naturally comparable to that of the iron pnictides, in which both the electron pockets near M and the hole pockets near Γ promote these two pairing components. Enhancement of pairing amplitudes near Mott transition The results for both classes of materials ( Figs 3c,d and 4 ) also show that the pairing amplitudes are larger when J 1 / D and J 2 / D are increased. This conclusion, in turn, leads to a general principle. To see this, we note that the exchange interactions increase as the Mott transition is approached from the insulating side ( cf. , Fig. 1 ) because of the reduction of the charge gap. At the same time, the renormalized bandwidth D is reduced as the Mott transition is approached from the metallic side. Correspondingly, at the boundary between electronic localization and delocalization, the ratios J 1 / D and J 2 / D will be maximized and so will the superconducting pairing amplitudes. Our results provide the understanding for some key experimental observations. Inelastic neutron-scattering experiments have shown that the exchange interactions in the alkaline iron selenides and iron pnictides have the same order of magnitude [16] . Further, as Fig. 1 illustrates, the alkaline iron selenides and iron pnictides have approximately the same doping concentration and similar degree of proximity to the Mott transition. Therefore, J 1 / D and J 2 / D are similar in the two materials. This leads to our key conclusion, namely, the two classes of iron-based superconductors have comparable pairing amplitudes and, by extension, comparable T c . It is instructive to contrast the situation here with KFe 2 As 2 . The latter system, with the Fermi surface containing only hole pockets [28] , represents another material lacking Fermi-surface nesting. However, it is strongly doped, with a hole doping of 0.5 per Fe. This extreme overdoping in KFe 2 As 2 means that the system is far away from the Mott transition-anchoring point discussed here and should, therefore, have considerably reduced pairing amplitudes. Experimentally, it indeed has a much smaller T c of about 3 K. For the alkaline iron selenides, our results show dominating A 1 g and B 1 g wave states in competition. Both have nearly isotropic and nodeless gaps on the electron pockets, and this is consistent with all existing measurements of the superconducting gap. Neutron-scattering experiments have identified a resonance associated with the superconducting state [29] . This is most readily understood in terms of a B 1 g wave pairing [29] , although it may also arise from an A 1 g channel once the effect of two iron ions per unit cell is taken into account [30] . On the other hand, ARPES experiments have suggested that the superconducting gap is nodeless on the faint electron pocket near the Γ point [30] , [31] . This appears to favour an A 1 g wave pairing [30] , [31] . Further experiments are needed to settle which of the two possible pairing channels operates in the alkaline iron selenides. For the iron pnictides, the dominance of A 1 g state in a large portion of the phase diagram is consistent with the sign-changing s ± paired state arising in both weak and strong-coupling approaches. Compared with the alkaline iron selenides, an important difference is that the pairing amplitude in the A 1 g channel is sizable ( Figs 3 , 4 ). This arises because the corresponding form factor, (cos k x +cos k y ), while negligible at the dominant electron Fermi surfaces located near the M points for the alkaline iron selenides, is large near the hole Fermi pockets around the Γ point in the case of the iron pnictides. The relevance of the A 1 g channel is important for understanding a possible strong momentum dependence or even the development of nodes in the superconducting gap; nodes arise on the electron Fermi pockets near the M points when the amplitude of the A 1 g component exceeds a threshold value compared with that of the coexisting A 1 g component. Indeed, experimentally, some iron pnictide superconductors show fully gapped behaviour, whereas others display properties that suggest the existence of nodes. The bad metal behaviour near the Mott transition also pertains to the relationship between magnetism and superconductivity in the alkaline iron selenides. For the vacancy-ordered parent insulating system (the so-called 245 phase), it causes the electronic excitations to have a large incoherent component; the latter gives rise to a large spin spectral weight even in the absence of any itinerant carriers, as have been observed by neutron-scattering experiments [15] , [16] . In superconducting compounds, there is direct evidence for a phase separation [32] between a superconducting component and the parent insulating anti-ferromagnetic part. The superconducting component is free of ordered vacancies [32] , suggesting a tetragonal 122 structure as we have used in our model. Our study here focuses on the pairing instabilities in the underlying metallic state of this component while taking advantage of its connection with the Mott-insulating phase in the overall phase diagram [33] discussed in the Supplementary Note 3 (and Supplementary Fig. S5 ) and evidenced by recent experiments [34] , [35] , [36] . It is worth emphasizing that the physical pathway linking the superconducting phase and 245 Mott-insulating phase involves varying both vacancy order and carrier concentration. Indeed, the existence of the multiple phases of the alkaline iron selenides suggests an overall, extended, parameter space in which the different phases can be connected. This is described in some detail in the Supplementary Note 3 and is in particular illustrated in Supplementary Fig. S5 . The details of this physical pathway is a distinct issue that is intriguing and important in its own right [33] , [34] , and other alkaline iron selenides such as KFe 1.5 Se 2 , with one vacancy per four iron sites [6] , [37] (and small carrier doping [34] , [38] ), and K 0.5 Fe 1.75 Se 2 , with one vacancy per eight iron sites [39] , may also be placed in this extended phase diagram. For the purpose of the present work, what is particularly pertinent is the clue these multiple phases have provided for the strength of the electron correlations. As described in the introduction and illustrated in Fig. 1 , the existence of the Mott-insulating phase in the 245 compound suggests not only that the underlying U / W is larger than U c / W in the vacancy-ordered alkaline iron selenides but also that U / W is below but close to U c / W in the iron pnictides. This proximity to the Mott transition allows for the present study on the pairing amplitudes in both classes of iron-based superconductors. Recently, superconductivity of around 50 K was reported in a single-layer FeSe film grown on SrTiO 3 substrate [40] . ARPES measurements [41] indicate that the Fermi surface consists of only electron pockets, similar to that of the alkaline iron selenides. Thus, it is instructive to model the single-layer FeSe film and compare its pairing properties with those of the other iron-based superconductors. We have thus studied the singlet superconductivity in a similar five-orbital t – J 1 – J 2 model for the single-layer FeSe film (see Methods), with an electron doping of 0.1 per Fe; we consider the role of the substrate as providing the structure that dopes this amount of electron carriers into the single-layer FeSe [42] , [43] . The results are shown in Supplementary Figs S4d and S7 . The pairing phase diagram of the single-layer FeSe is comparable to those for both alkaline iron selenides and iron pnictides, and so are the overall pairing amplitudes. By showing that pairing amplitudes are similar for the iron chalcogenides and pnictides in spite of their drastically different Fermi surfaces, our results uncover a universality in the existing and emerging iron-based high-temperature superconductors with very diverse materials and Fermi-surface characteristics. Moreover, our demonstration, that the pairing amplitudes increase with the ratio of the short-range spin exchange energy to the renormalized kinetic energy, reveals an important principle. Namely, superconductivity is optimized at the border between itinerancy and electronic localization. This principle should apply beyond the context of iron pnictides and chalcogenides, and is expected to guide the search for superconductors with even higher transition temperatures. Multi-orbital t – J 1 – J 2 model We describe the methods used in our study of the phase diagram for the singlet superconducting pairing of five-orbital t – J 1 – J 2 models, described as H = H t + H J . Here, H t and H J , respectively, correspond to the fermion hopping and the J 1 – J 2 exchange Hamiltonians. Two such models are considered. The difference in the fermiology of the alkaline iron selenides and iron pnictides are specified via the kinetic part H t , and we have chosen the tight-binding parameters by fitting the band dispersions obtained from density functional calculations. The short-range anti-ferromagnetic exchange interactions in H J drive the singlet pairings. We have chosen the same exchange-coupling constants J 1 , J 2 for each orbital, and have performed a mean-field decoupling of the exchange part in the pairing channel. Each orbital contributes four pairing amplitudes Δ a , α , which are, respectively, given by , α , , α , , α , d xy , α , where α =1,...,5 labels the orbitals; these amplitudes are related to their real-space counterparts, Δ e , α =‹ c iα ↑ c i + e α ↓ − c iα ↓ c i + e α ↑ ›/2. We have minimized the free energy to find the self-consistent solution for the 20 pairing amplitudes. We now expound on these in some detail. Our five-orbital t – J 1 – J 2 model arises from an expansion of the five-orbital Hubbard model with respect to the Mott transition point (the ‘ w -expansion’) [20] . The Hamiltonian for the model is given by where creates an electron at site i , with orbital index α and spin projection s ; μ is the chemical potential and the hopping matrix. The orbital index α =1, 2, 3, 4 and 5 respectively, correspond to five 3 d orbitals 3 d xz , 3 d yz , , 3 d xy and of iron. The n.n. (‹ ij ›) and n.n.n. (‹‹ ij ››) exchange interactions are, respectively, denoted by and . The spin operator and the density operator , with representing the Pauli matrices. For the calculation in these five-orbital models, we have considered the effects of the fermion no double-occupancy constraints as being implicitly accounted for by the reduction of the effective bandwidth D . We expect that this treatment does not affect the results qualitatively. We have verified this expectation for a two-orbital model by explicitly keeping track of the occupancy constraints. This is described in some detail in the Supplementary Note 1 ; Supplementary Methods and Supplementary Fig. S3 . As shown there, the phase diagram and pairing amplitudes are insensitive to this when the exchange interactions are measured with respect to the renormalized bandwidth D . In a previous study of a multiorbital t – J 1 – J 2 model for iron pnictides [21] , it has been demonstrated by three of the present authors that the dominant pairing symmetry is governed by the intraorbital exchange interactions, and the consideration of the orbitally off-diagonal exchange interaction only introduces quantitative modifications of the phase diagram. Therefore, to keep the analysis simple, we will consider the orbitally diagonal exchange couplings and . To consider a pure superconducting phase, we will study here the case with the 122 tetragonal symmetry (see Supplementary Note 3 for further discussions). To describe the fermiology, we use a tetragonal symmetry-preserving tight-binding model, involving all five 3 d orbitals of iron. In the momentum space, the 5 × 5 tight-binding matrix, and its eigenvalues will be, respectively, denoted by and E j , k . The total number of electrons is determined by the chemical potential and the dispersion relations, according to , and carrier doping δ =| n −6|. The tight-binding parameters are fixed by fitting the band structure obtained from the local density approximation (LDA) calculation. The details of the tight-binding parametrization for iron chalcogenides and the associated band dispersions are discussed below, in the next subsection. For (K,Tl) 1− x Fe 2− y Se 2 , the band dispersions correctly produce the electron pockets near the M points, as illustrated in Fig. 2a for K 1− x Fe 2− y Se 2 . The electron- and hole-like Fermi pockets obtained from a similar five-orbital tight-binding model of iron pnictides [27] are shown in Fig. 2b to contrast the fermiology of the two materials. The fermiology of Tl 1− x Fe 2− y Se 2 is shown below, in Supplementary Note 2 and Supplementary Figs S1 and S2 , which again consists of only electron pockets. We note that ARPES experiments [8] , [9] , [10] have suggested that very weak electron-like pockets may also exist near the Γ points. Unlike their hole counterpart in the iron pnictides, these electron pockets have very small spectral weight and are expected to have at most a secondary role in driving superconductivity. Details of tight-binding parametrization For the five orbital, tetragonal symmetry preserving tight-binding model, we adopt the parametrization method of Graser et al. [27] We have fitted the LDA band structure with the band dispersion found from the tight-binding model to determine the hopping parameters. For (K,Tl) 1− x Fe 2− y Se 2 , we have performed calculations with two different sets of hopping parameters (see Supplementary Tables S1 and S2 ). These two sets, respectively, were derived from fitting the LDA results for KFe 2 Se 2 and TlFe 2 Se 2 ; see Supplementary Fig. S1 . For iron pnictides, we use the tight-binding parameters of ref. 27 . In Figs 2a and 3a , we have shown the electron pockets and pairing phase diagram for the band structure corresponding to K 1− x Fe 2− y Se 2 . In Supplementary Fig. S1 , we provide the band dispersions for both tight-binding models and also show the electron pockets derived from Tl 1− x Fe 2− y Se 2 . Spin singlet-pairing states We first consider degenerate pairing states in the absence of kinetic energy. The spin singlet, intraorbital-pairing operators are defined as Δ e , α ≡Δ e , αα =‹ c iα ↑ c i + e α ↓ − c iα ↓ c i + e α ↑ ›/2, where . Two types of pairing states , respectively, denoted as and states with momentum space form factors =cos k x +cos k y ; =cos k x −cos k y arise because of the n.n. exchange interaction, and they are energetically degenerate in the absence of kinetic energy. Similarly, the n.n.n. exchange gives rise to two degenerate pairing states , respectively, denoted as and d xy states, with momentum space form factors =cos( k x − k y )+cos( k x + k y ), g xy , k =cos( k x − k y )−cos( k x + k y ). A strong magnetic frustration, characterized by , leads to an enhanced degeneracy among the four paired states. The kinetic energy term lifts most of these degeneracies. In the strong frustration regime ( ), it leaves a quasi-degeneracy among a reduced set of pairing states. To study the full problem, we perform a mean-field decoupling [21] , [44] of the exchange interaction terms. We introduce four complex singlet-pairing amplitudes for each orbital and write the following 5 × 5 pairing matrix , where and the index a corresponds to , , and d xy symmetries. In the subspace of xz and yz orbitals, which transform as a doublet under the tetragonal point group operations, there are the following four classes of intraorbital-pairing states for an orbitally diagonal J 1 – J 2 model: (i) ; (ii) ; (iii) ; and (iv) . The eight pairing amplitudes and so on are obtained as linear combinations of and , which are in turn linear combinations of Δ e ,11 and Δ e ,22 . Mixed-symmetry-pairing states breaking time-reversal symmetry The admixed states II and III of Fig. 3a,b break time-reversal symmetry and have the form A 1 g + iB 1 g . In regions II and III, the A 1 g components are, respectively, cos k x cos k y and (cos k x +cos k y ). In contrast to the pnictides, the pairing phase diagram of 122 chalcogenides has a region IV, which is of purely B 1 g character even at zero temperature. The time-reversal symmetry breaking in region II is because of quasi-degeneracy between and pairings induced by strong magnetic frustration. On the other hand, the quasi-degeneracy between and pairings in region III arises because of bandwith suppression. These mixed-symmetry-pairing states are expected to be relevant only at sufficiently low temperatures. Generalizations of the models The pairing phase diagrams, shown in Fig. 3a,b , have been determined by assuming orbitally diagonal exchange couplings J 1 and J 2 . The interorbital exchange couplings do not qualitatively modify the phase diagram. The interorbital couplings introduce some subdominant components to A 1 g and B 1 g regions, while leaving the competition between A 1 g and B 1 g pairing symmetries intact. For example, an interorbital second neighbour coupling between xz and yz orbitals gives rise to interorbital d xy (sin k x sin k y ) component, which is a part of A 1 g pairing. Similarly, we can also consider further neighbour intraorbital exchange couplings. For example, the third neighbour anti-ferromagnetic exchange-coupling J 3 does not change the competing pairing channels; however, it introduces subdominant A 1 g (cos 2 k x +cos 2 k y ) and B 1 g (cos 2 k x −cos 2 k y ) components. Therefore, the phase diagram obtained from an orbitally diagonal J 1 – J 2 model is generic and robust. We also note that an extended J 1 – J 2 model [16] , [45] , with ferromagnetic n.n. coupling, defined on a modulated square lattice, has been used to explain the block spin anti-ferromagnetic order. Although this is believed to reflect the modulation to the exchange interactions that exists only in the presence of ordered vacancies [45] , [46] , it is interesting to consider the effect of a ferromagnetic J 1 . The latter will suppress the B 1 g pairing and increase the A 1 g region. We stress that the A 1 g – B 1 g competition described earlier is the feature of the paramagnetic state, which is devoid of vacancy order and should have an anti-ferromagnetic J 1 . Finally, higher-spin interactions such as a biquadratic term can also be incorporated in the model. These interactions will generate contributions to the free energy that are of higher order in the pairing amplitudes. Therefore, they will not significantly affect the competition among the different pairing channels. Estimate of the superconducting energy gaps Our results allow an order-of-magnitude estimate of the pairing energy gaps for the alkaline iron selenides and optimally doped iron pnictides. For both alkaline iron selenides and iron pnictides, the energies of the zone-boundary magnetic excitations are on the order of 200 meV, which imply that the effective exchange interactions are on the order of 20–50 meV [16] , [47] . This specifies the order of magnitude of the parameters J 1 and J 2 in our model, although they are for individual orbitals. Our calculated values for the pairing amplitudes Δ ( Fig. 3c,d ) then imply that the corresponding pairing gaps, , appropriately weighted over the different orbitals, will be on the order of 10 meV. This is compatible with what have been inferred from the ARPES and tunnelling measurements [8] , [9] , [10] , [32] . Pairing for the single-layer FeSe film We consider the spin singlet pairing of a five-orbital t – J 1 – J 2 model for the newly discovered single-layer FeSe film [40] . Recent experiments [40] , [41] suggest that superconductivity arises from the FeSe layer but not from the FeSe/SrTiO 3 interface. Hence, we study, using density functional theory, the electronic structure of a single-layer FeSe without including a substrate. We then use a five-orbital tight-binding parametrization described earlier in the Methods section to fit the density functional theory bandstructure. The best-fitted tight-binding parameters are listed in Supplementary Table S3 . Supplementary Figure S6a shows the bandstructure of the tight-binding model with these parameters. We have fixed the Fermi energy so that the electron doping is 0.1 per Fe, which is close to the value of 0.09 per Fe determined by ARPES measurement [41] . As shown in Supplementary Fig. S6b , the calculated Fermi surface comprises electron pockets only, which is consistent with the ARPES results [41] . The overall bandwidth of this model is somewhat larger than that of K 1− x Fe 2− y Se 2 , suggesting the electrons are less correlated in the single-layer FeSe than in alkaline iron selenides. This is consistent with the weaker mass renormalization observed in the single-layer FeSe film [41] . Given these tight-binding parameters for the single-layer FeSe, the corresponding five-orbital t – J 1 – J 2 model is specified as described earlier in the Methods section. We again consider spin singlet pairing. Supplementary Figure S7 shows the pairing phase diagram and pairing amplitudes in several channels. Both phase diagram and strength of the pairing amplitudes are similar to those of alkaline iron selenides K 1− x Fe 2− y Se 2 and Tl 1− x Fe 2− y Se 2 . How to cite this article: Yu, R. et al. Superconductivity at the border of electron localization and itinerancy. Nat. Commun. 4:2783 doi: 10.1038/ncomms3783 (2013).